Somatic mutations in arachidonic acid metabolism pathway genes enhance oral cancer post-treatment disease-free survival The arachidonic acid metabolism (AAM) pathway promotes tumour progression. Chemical inhibitors of AAM pathway prolong post-treatment survival of cancer patients. Here we test whether non-synonymous somatic mutations in genes of this pathway, acting as natural inhibitors, increase post-treatment survival. We identify loss-of-function somatic mutations in 15 (18%) of 84 treatment-naïve oral cancer patients by whole-exome sequencing, which we map to genes of AAM pathway. Patients ( n =53) who survived ≥12 months after surgery without recurrence have significantly ( P =0.007) higher proportion (26% versus 3%) of mutations than those who did not ( n =31). Patients with mutations have a significantly ( P =0.003) longer median disease-free survival (24 months) than those without (13 months). Compared with the presence of a mutation, absence of any mutation increases the hazard ratio for death (11.3) significantly ( P =0.018). The inferences are strengthened when we pool our data with The Cancer Genome Atlas (TCGA) data. In patients with AAM pathway mutations, some downstream pathways, such as the PI3K–Akt pathway, are downregulated. The arachidonic acid (AA) metabolism pathway, hereinafter referred to as the AAM pathway, a key inflammatory pathway involved in cellular signalling, has been implicated in diverse human cancers [1] . This pathway generates genotoxic agents, such as, reactive oxygen species, peroxides, free organic radicals and aldehydes that promote tumorigenesis [2] , [3] . AA, a common dietary fatty acid stored in cell membranes and in extracellular microenvironment, is released in response to extracellular stimuli and mobilized by phospholipase A2 (PLA2) and converted to prostaglandins, hydroperoxyeicosatetraenoic acids and epoxyeicosatrienoic acids by the action of cyclooxygenases (COXs), lipoxygenases (LOXs) and cytochrome P450 (CYP) epoxygenases, respectively [1] , [4] , [5] . AAM pathway promotes tumour progression by activating major mitogenic signalling pathways, including PI3K, MAPK and Jun kinase [6] , [7] , [8] . AA metabolism cascade is involved in head and neck squamous cell carcinoma (HNSCC) [9] , [10] , [11] , [12] , particularly in oral squamous cell carcinoma (OSCC) [13] . OSCC is the eight most common cancer in the world and constitutes a major cancer burden predominantly among males in India [14] . In most (60%) Indian OSCC patients, the gingivo-buccal (GB) area—comprising the buccal mucosa, the retromolar trigone and the lower gum—is affected, while in Western patients the tongue is predominantly (65%) affected [15] , [16] . Most OSCC-GB patients present at advanced stages (stages III and IV), have a very high locoregional failure rate and their rate of mortality has remained high and unchanged for over three decades despite the best multimodal treatment [17] , [18] . Recently, we [14] and others [19] , [20] , [21] , [22] have identified, by exome sequencing, somatic driver mutations and key pathways in HNSCC, which show that OSCC is primarily driven by mutations in TP53 , FAT1 , CASP8 , NOTCH1 and USP9X genes; these genes are tumour suppressors and, therefore, difficult to target by drugs. Several members of AAM pathway were reported to overexpress in different cancers and modulate cancer progression [23] , [24] . Median disease-free survival (DFS) in cholangiocarcinoma patients was significantly better in patients with low levels of 5-LOX or COX-2 expression than those with high levels [25] . Lipid autacoids that are CYP-derived metabolites of AA appear to be involved in cancer either by regulating cell-autonomous tumour survival and growth or by modulating stromal processes, such as angiogenesis and inflammation that can support tumour progression [26] . Recent studies [12] , [27] , [28] , [29] have reported that inhibitors of different components of the AAM pathway show promising results in the treatment of various human cancers including premalignant lesions of HNSCC [30] . Synthetic inhibitors of CYP significantly reduced tumour size in intracranial glial tumours and prolonged survival of treated rats [31] . A clinical trial ( http://clinicaltrials.gov/ct2/show/NCT00620139 ) is underway to study the proximal effects of concurrent chemotherapy on the expression of potential molecular targets on the AAM pathways in HNSCC. Since AAM pathway inhibitors hold promise for cancer treatment, including prolonging post-treatment survival [25] , [31] , we hypothesize that non-synonymous somatic mutations in genes of the AAM pathway act as natural inhibitors of the pathway and enhance post-treatment survival probability of OSCC-GB patients. We analyse the somatic mutation profile of genes on the AAM pathway in OSCC-GB patients and discover robust evidence in support of the hypothesis. Case description, human papillomavirus infection and exome sequencing Tumour and blood samples from 110 patients diagnosed with OSCC-GB were collected, with informed consent, at the time of surgical excision. Three patients who died of causes other than cancer were excluded. Twenty-three living patients for whom the follow-up period was <12 months were also excluded. 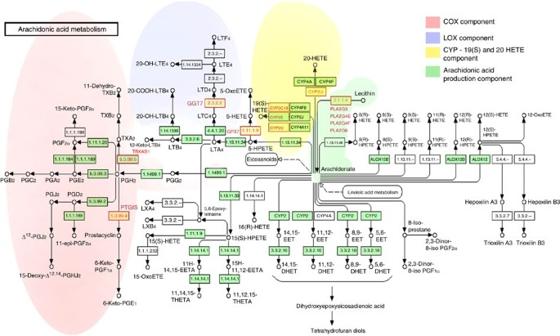Figure 1: Somatically mutated genes in AAM pathway among patients with OSCC-GB. Mutations in AAM pathway genes were mapped on the KEGG pathway map. Genes in the red boxes are those with somatic mutations and genes in green boxes are without any somatic mutation. The remaining patients ( n =84) included in this study (see Supplementary Table 1 , for their characteristics) were categorized into two subgroups based on whether (SRV12; n =53) or not (N-SRV12; n =31) they survived for at least 12 months after surgery without recurrence. (Varying the period of survival by ±6 months to define the subgroups did not change inferences; results not shown.) Survival and recurrence data were collected by following up the treated patients from the date of surgery to 39 months—the longest observed duration of survival. Median DFS was 14 months. In the total cohort, the percentage of patients who were alive for >1 year was 63%, >2 years was 33% and >3 years was 2%. Recurrence at the primary site was confirmed in 40 out of 84 patients (47.6%). Human papillomavirus infection (HPV) infection, all with high-risk subtypes (16 and 18), was detected in 20% of patients. 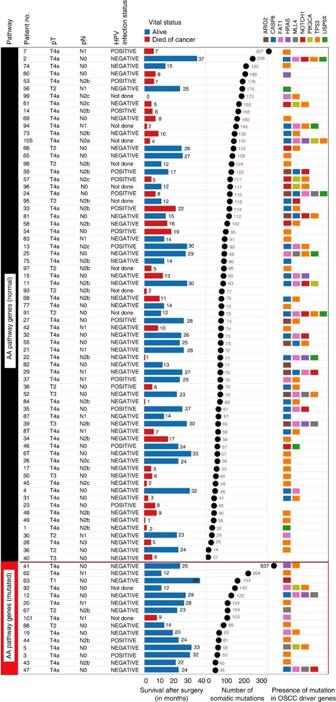Figure 2: Clinical, pathological and molecular features of patients without (norAA) and with (mutAA) mutations in genes of the arachidonic acid metabolism (AAM) pathway. In the vertical panel, for each patient, the tumor stage (pT), local lymph node metastasis status (pN), HPV infection status, vital status, total number of somatic mutations and mutation status in known OSCC driver genes are shown. These data have been arranged by groups of patients with or without mutations in genes of the AAM pathway in increasing order of the total number of mutations observed in each patient. Colour coding schemes for vital status and driver gene mutation status are indicated on top of the figure. Tumour-normal pairs of the 84 patients were sequenced at a mean depth of 44.94±1.83 (details in Supplementary Table 2 ). 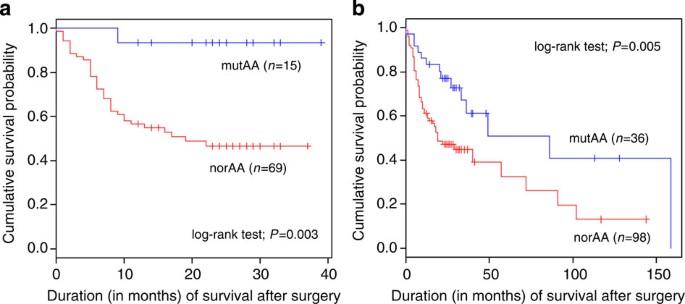Figure 3: Kaplan–Meier probability distributions of disease-free survival. (a) Subgroups of OSCC-GB patients, with (mutAA) or without (norAA) loss-of-function mutations in genes of the arachidonic acid metabolism pathway; and (b) OSCC-GB patients included in this study pooled with those included in The Cancer Genome Atlas (TCGA) study. In addition, exome sequence data were also generated for 17 of the 23 patients who were alive for a period of <12 months (short follow-up cases); their mutation profiles are given in Supplementary Table 3 . Molecular data of these patients were not included in the survival analysis. Longer OSCC-GB survivors have larger number of AAM mutations Loss-of-function somatic mutations in the coding regions of one or more of the 63 AAM pathway genes (KEGG pathway id—hsa00590) were detected in 15 (18%) of the 84 tumours ( Table 1 ). A significantly ( P =0.007) higher proportion (26%) of patients who survived for >12 months without recurrence (SRV12 subgroup) possessed somatic mutations in one or more genes compared with those (N-SRV12 subgroup) who died within 12 months after surgery (3%). The median duration—24 months—of post-treatment survival of patients in the SRV12 subgroup was significantly ( P <0.001) higher than patients in the N-SRV12 subgroup for whom the median duration was 6 months. Table 1 List of genes of the AA metabolism pathway with somatic loss-of-function mutations among 15 OSCC-GB patients and other relevant details. Full size table In addition, genome-wide copy number alteration analysis revealed that there was no statistically significant difference (Fisher’s exact P value=0.623) in the proportion of patients with CN loss in genes of the AAM pathway among those who survived for >12 months (14%) compared with those who did not survive for this length of time (8%; Supplementary Table 4 ). Mutational profiles of AAM pathway in oral cancer The AAM pathway is partitioned into four major sub-components, (I) AA production from membrane phosopholipids by phospholipases and generation of various tumour-inducing inflammatory molecules, like prostaglandins, through metabolism of AA by the action of various (II) COX, leukotrienes by the action of (III) LOX enzymes, and production of several hydroxyeicosatetraenoic acids (HETEs) and epoxyeicosatrienoic acids by the action of (IV) P450 epoxygenase enzymes [32] . Fifteen non-synonymous somatic single-nucleotide substitutions were identified in 10 genes of the pathway; of which 13 (86%) were predicted to be missense and 2 (14%) were nonsense mutations ( Table 1 ). No somatic insertions or deletions were detected in these genes. These somatic mutations were restricted to specific sub-components of the AAM pathway, which were (a) AA production (four mutated genes— PLA2G3 , PLA2G4E , PLA2G4F , PLA2G6 ), (b) prostaglandin production (mutations in prostacyclin synthase ( PTGIS) and TBXAS1 ), (c) leukotriene production (one mutated gene, GGT7 ), (d) 5, 19 and 20-HETE production (two mutated genes, CYP2C19 and CYP2U1 ; see Fig. 1 ). Two or more samples were discovered to harbour somatic mutations in four genes— GGT7 , PTGIS , CYP2U1 and GPX7 . GGT7 that are involved in the production of potent cancer inducer LTD4 leukotriene [1] , [33] . The enzyme PTGIS catalyses the conversion of prostaglandin H2 ( PGH2 ) to prostaglandin I2 ( PGI2 ). PGI2 promotes cancer growth by activating peroxisome proliferator-activated receptor δ and increases the expression levels of the pro-angiogenic factor vascular endothelial growth factor [34] , [35] . CYP2U1 is a hydroxylase that metabolizes AA and produces 20-HETE synthesis, which is associated with the growth of cancer cells in vitro and in vivo and is also upregulated in various human cancers [36] . Other mutated genes of this pathway are known to aid tumour growth. Of these, GGT7 and PLA2G3 harbour nonsense mutations. Figure 1: Somatically mutated genes in AAM pathway among patients with OSCC-GB. Mutations in AAM pathway genes were mapped on the KEGG pathway map. Genes in the red boxes are those with somatic mutations and genes in green boxes are without any somatic mutation. Full size image Patients with AAM pathway mutations survive longer The median duration of DFS without recurrence was 14 months (details on Fig. 2 ). The proportions of patients at advanced stages (T3 or T4) of tumour, lymph node involvement, smoking and chewing habits, alcohol intake, perineural invasion, and bone and skin involvement were not significantly different ( P >0.05) between the non-mutated AA (norAA) and mutated AA (mutAA) subgroups of patients. During the follow-up period, a significantly higher proportion ( P =0.003) of patients (35 patients; 50.7%) in the norAA subgroup died of cancer than in the mutAA subgroup (one patient; 6%). Mutation in any gene of the AA metabolism was associated with a significant ( P =0.003) increase in the median duration of DFS; median durations of DFS in mutAA patients was 24 months, while in norAA patients was 13 months. The Kaplan–Meier survival probability distributions are given in ( Fig. 3a ). Figure 2: Clinical, pathological and molecular features of patients without (norAA) and with (mutAA) mutations in genes of the arachidonic acid metabolism (AAM) pathway. In the vertical panel, for each patient, the tumor stage (pT), local lymph node metastasis status (pN), HPV infection status, vital status, total number of somatic mutations and mutation status in known OSCC driver genes are shown. These data have been arranged by groups of patients with or without mutations in genes of the AAM pathway in increasing order of the total number of mutations observed in each patient. Colour coding schemes for vital status and driver gene mutation status are indicated on top of the figure. Full size image Figure 3: Kaplan–Meier probability distributions of disease-free survival. ( a ) Subgroups of OSCC-GB patients, with (mutAA) or without (norAA) loss-of-function mutations in genes of the arachidonic acid metabolism pathway; and ( b ) OSCC-GB patients included in this study pooled with those included in The Cancer Genome Atlas (TCGA) study. Full size image This significant increase in DFS in the mutAA subgroup is not because of the effect of plausible covariates. Recent studies have revealed that (i) intratumour heterogeneity was higher in poor-outcome classes of HNSCC [37] , and (ii) HPV infection had a favourable outcome among HNSCC patients [38] , [39] . HPV infection rates were similar ( P =0.72; 21.7% in norAA, 13% in mutAA), the mean number of somatic mutations were similar ( P =0.66, t -test of equality of means 95.8±12.5 in mutAA, 89.9±5.6 in norAA. (Two outlier patients with large numbers of somatic mutations, 307 and 622, were excluded from these calculations.) These results were also validated by a multiple regression analysis with DFS as the dependent variable and with independent variables; (a) total number of somatic mutations, (b) whether any gene of AAM pathway was mutated and (c) whether there was HPV infection. The P values corresponding to the three independent variables were, respectively, 1.0, 0.004 and 0.849. Thus, DFS is associated only with mutation in any gene, but not with the total number of mutations or HPV infection status. Compared with the presence of a AAM pathway mutation, the absence of any mutation on this pathway significantly ( P =0.018) increased the hazard ratio for death (11.3; 95% confidence interval 1.5–84.5) even when considered jointly with other variables (age, sex, tumour stage, lymph node involvement and total number of somatic mutations, in a Cox’s proportion hazards model ( Supplementary Table 5 ). Driver gene profiles are similar in mutAA versus norAA subgroups The mutAA subgroup had similar mutation profiles in HNSCC/OSCC-GB driver genes— TP53 , CASP8 , FAT1 , NOTCH1 , USP9X , ARID2 , HRAS , MLL4 and PIK3CA —as the norAA subgroup ( Fig. 2 ). The total number of mutations per patient in these genes was not significantly different ( P =0.36) between the norAA (2.39±0.19) and mutAA subgroups (2.0±0.33). Every patient in the mutAA subgroup had at least one somatic mutation in an important OSCC driver gene. The proportions of patients with a somatic mutation in OSCC-GB driver genes were similar in both the subgroups ( Supplementary Table 6 ), except ARID2 and USP9X , which were mutated only in the norAA subgroup (13%). The percentage of patients with somatically mutated MLL4 in the mutAA subgroup (26%) was significantly higher ( P =0.01; test of proportions) than that in the norAA subgroup (6%), but the mean number of somatic mutations were similar ( P =0.58) in both the subgroups (4.86 in mutAA and 4.31 in norAA). The average mutation rates in DNA repair genes [40] — ATM , ATR, BRCA1 , BRCA2 , CHEK1 , CHEK2 , FANCF , MLH1 , MSH2 , MDC1 , PARP1 and RAD51 —were similar ( P >0.05) in both the subgroups. Further, the proportions of patients with mutations in genes in each mitogenic drug targetable pathway as defined in the KEGG database, namely PI3K–AKT, MAPK, JAK–STAT and WNT signalling, were similar in both the subgroups ( P values for all four tests of equality of proportions were >0.05; Supplementary Fig. 1 ). These results show that the survival advantage enjoyed by patients with somatic mutations in genes of the AAM pathway is not due to confounding factors. Pooling of TCGA data strengthens inferences Data of patients with cancer of oral cavity and buccal mucosa ( n =50) in the TCGA-HNSCC data set ( https://www.synapse.org/#!Synapse:syn1446094 ) were mined for the presence of somatic mutations in AAM pathway genes. In the TCGA-OSCC subset, 21 patients (42.0%) had one or more loss-of-function somatic mutations in genes of the AAM pathway ( Supplementary Table 7 ). In the pooled set of OSCC-GB patients included in the present ( n =84) and the TCGA studies ( n =50), the presence of a mutation in any gene of the AAM pathway was significantly associated with increased DFS (log-rank test; P =0.005). The Kaplan–Meier survival probability distributions are given in Fig. 3b . These inferences also hold if the data on all HNSCC patients included in the TCGA study ( n =224) are pooled with the data on OSCC-GB patients ( n =84) of the present study. In the TCGA-HNSCC subset, 59 patients (26.0%) had one or more loss-of-function somatic mutations in genes of the AAM pathway ( Supplementary Data 1 ). The total number of mutations was not significantly associated with DFS in the pooled data set either for OSCC-GB ( P =0.543) or HNSCC ( P =0.905). (Information on HPV infection was not available in the TCGA data set.) In the pooled ( n =308) data set, patients with a mutation in any AAM pathway gene ( n =74) had significantly elevated duration of median DFS (39 months) compared with those ( n =234) without mutations (29 months; log-rank test; P =0.007). The Kaplan–Meier survival probability distributions for pooled data are given in Supplementary Fig. 2 . PI3K–Akt cascade is downregulated in mutAA patients Functional proteomics data were also available, in the RRPA data set of the TCGA study, on the HNSCC patients of TCGA considered in the present study. Protein levels between patients with ( n =57) or without ( n =167) mutated AAM pathway genes were analysed. Differences of protein levels of five genes were found to be statistically significant ( P <0.05) between these two groups. Out of these five genes, four genes are known oncogenes (AXL, FN1, MACC1 and IRS1) [41] , [42] , [43] , [44] , [45] , which produce significantly low levels of the proteins in patients with mutation in AAM pathway ( Supplementary Fig. 3a ). Three (AXL, FN1 and IRS1) of these four genes are on the KEGG PI3K–Akt pathway [45] , [46] . Further, among all transcription factors, STAT3 and NFKB1 were found to have the lowest levels of phosphorylation among patients with mutations in AAM pathway genes; the levels among patients without mutations were significantly ( P <0.05) higher ( Supplementary Fig. 3b ). Activation of these two transcription factors are known to be mediated by the PI3K–Akt pathway [47] , [48] . The PI3K–Akt pathway is known to be activated by AA metabolism pathway end-products [6] , [49] in cancer. PI3K–Akt pathway is a well-known driver of HNSCC [50] , [51] . Compared with the patients without mutation in AAM pathway genes, those with mutation have low protein levels of oncogenes associated with the PI3K–Akt pathway. The low levels of phosphorylation of transcription factors STAT3 and NFKB1, activations of which are mediated by this pathway, also provides indirect support that PI3K–Akt pathway is downregulated among patients with mutated AAM pathway. These are likely explanations of the higher survival benefits observed in HNSCC patients with mutated AAM pathway. Genes on the AAM pathway are known to overexpress and activate other pathways that promote cancer [1] , [52] . Targets on this pathway have already been intensively studied in other diseases, such as cardiovascular diseases and pain, providing an opportunity for repurposing of drugs already in clinical development to new indications [53] . AA is the central transducer molecule generated from membrane phospholipids by phospholipase enzymes and converted to biologically active tumorigenic eicosanoids by COX, LOX and CYP enzymes. Various genes in this pathway were found to be mutated in a subgroup of patients in this study. The study among Indian OSCC-GB patients has revealed that (a) overall rates and profiles of somatic mutations are similar in the two subgroups of patients with (mutAA) and without (norAA) mutations in genes of the AAM pathway, and (b) the mutAA subgroup of patients harbours mutations in components of AA production and those that induce tumour progression via COX, LOX and CYP enzymes. We have identified missense mutations in four PLA2s family of genes, belonging to groups III, IV and VI, which are involved in the production of AA from membrane phospholipids. Most human PLA2 enzymes overexpress in a proportion of tumours derived from diverse organs including HNSCC [54] , [55] , [56] and inhibition of PLA2 alters cancer cell growth and death in vitro [57] . Combination therapy of PLA2 group VI inhibitor and paclitaxel for xenograft model of ovarian cancer have shown promising results [58] . We have detected two mutations in PTGIS and one mutation in thromboxane A synthase 1 ( TBXAS1 ) gene. A recent study [59] has suggested that PTGIS or TBXAS1 may be better therapeutic targets than the most studied and validated target cyclooxygenase-2 ( PTGS2 ) gene in breast cancer. Prostaglandin-targeted therapies (for example, COX inhibitors) are presently under investigation for chemoprevention of a variety of cancers including lung, colorectal and breast cancers [60] . We have discovered two genes in the LOX pathway— GGT7 and GPX7 —to be mutated. Increased LOX expression levels have been observed in a broad range of cancers, including breast, pancreatic, prostate, lung, urinary bladder, leukaemia and colon cancer [53] . Inhibitors against members of LOX pathway have chemopreventive effects against various cancers [61] , [62] , [63] . Germline variant genotypes in 12-LOX gene reduce the risk of rectal cancer by 33% (ref. 64 ). Wild-type COX and LOX pathway genes elicit the most potent inflammatory signalling molecules; therefore, blocking these pathways show additive effect in colon cancer cells [65] . We detected mutations in CYPC219 gene, which is known to overexpress in hepatocellular carcinoma in Chinese patients [66] , and also in CYP2U1 gene, which is overexpressed in colorectal and ovarian cancers [67] , [68] . Combined target inhibition of various combinations of COX, LOX, CYP enzymes as well as inhibition of AA metabolites are effective in human oesophageal, colon, breast and skin cancer [1] . Among the mutAA subgroup of patients, the median period of DFS is nearly double of that for the norAA subgroup of patients, which is significant (log-rank test; P =0.003). Further, only 6% patients of the mutAA subgroup died of cancer in contrast to 50.7% of norAA subgroup. These differences were not due to an increase in overall mutation frequency or frequency of HPV infection in the mutAA subgroup, nor even due to statistically significant differences with norAA subgroup in profiles of tumour grade, stage and lymph node involvement or of mutation frequencies in the major genes that drive OSCC-GB [14] . Our data combined with HNSCC data of the TCGA study showed that these are globally valid observations. Functional proteomics data revealed that indeed patients with AAM pathway mutations have significantly low protein levels of known oncogenes and low phosphorylation status of nuclear transcription factors, which play critical roles in the PI3K–Akt cascade. PI3k–Akt pathway is a known driver of HNSCC. Downregulation of this cascade in patients with mutated AAM pathway is congruent with their observed higher DFS and are likely to be the explanatory factors. Our results provide the definitive inference that presence of mutations in genes of AA metabolism pathway may be used as a prognostic marker of survival after treatment of GB oral cancer. Ethics approval and informed consent Institutional Ethics Committees of the Advanced Centre for Treatment, Research and Education in Cancer (ACTREC) and the National Institute of Biomedical Genomics (NIBMG) approved this study. Voluntary informed consent was obtained from each participant. Patient description Blood and tumour specimens were collected at surgical excision, from 110 treatment-naïve OSCC-GB patients, who underwent a comprehensive staging, curative resection, post-operative radiotherapy±chemotherapy and follow-up at ACTREC. Only patients with concordant histologic diagnoses by two independent and experienced histopathologists, who followed the WHO guidelines, were recruited into this study. Each patient was also followed up every month after surgery. At each follow-up, clinical checks of the primary site and relevant nodes were carried out for recurrence, and a verbal reporting of the health status was obtained from the patient. Clinical detection of recurrence was confirmed by histopathology. We have reported only cancer-specific deaths. Patients who died of causes other than cancer were excluded from the analyses. DFS time was estimated as the maximum follow-up period during which a patient remained free of OSCC after treatment. Subsequently, OSCC may have recurred in the patient or the patient may have died of other causes. DNA isolation, exome sequencing, genotyping and HPV assay DNA isolation, determination of HPV infection status—exome sequencing using three orthogonal technology platforms and whole-genome Illumina SNParray genotyping were done as described previously [14] . In brief, for exome sequencing, about 62 Mb of coding region of the human genome was captured using Illumina Tru-Seq exome enrichment kit and sequenced using Illumina Hiseq 2000. DNA samples were also captured for ~26 Mb of coding region by using Nimblegen SeqCap EZ and sequenced using Roche GS-FLX platforms to verify variants identified from the Illumina study. In addition, mutated variants from outside of the Nimblegen ~26 Mb capture region were verified using the Ion Torrent platform. Each blood and tumour exome library was sequenced at a minimum depth of 25 × and 35 × , respectively. Somatic mutation and copy number alteration determination, and verification Sequence data obtained using HiSeq-2000 were demultiplexed and FASTQ files were generated by CASAVA v1.8.2 (Illumina). FASTQC Ver. 0.10.1 ( http://www.bioinformatics.babraham.ac.uk/projects/fastqc/ ) was used to quality-check sequence data, using default parameters. Sequence reads with >10% N-bases were filtered and removed. Sequence reads with average quality value <20 were also removed. Filtered sequence reads were mapped to human genome reference sequence (hg19 with decoy sequence; ftp://ftp.1000genomes.ebi.ac.uk/vol1/ftp/technical/reference/phase2_reference_ assembly_sequence/) using BWA v0.6.1 with –q 15, −l 32 as arguments and SAM files were generated. Reads that mapped to decoy segments of the reference sequence and those that multiple mapped to various locations were removed from further analysis. Finally, unmapped and duplicate reads were filtered out using programs written by us and PICARD v1.60 ( http://picard.sourceforge.net ). GATK v. 1.4. was used for base quality recalibration, local realignment around indels using known single-nucleotide polymorphisms. Alignment SAM files were converted to BAM files using Samtools 0.1.12a. BAM files were converted to pileup format by SAMtools ( http://samtools.sourceforge.net/ ) for variant calling. Somatic variants were called using a base-by-base caller [14] . High confidence variants were identified using the following criteria, (i) variant base quality value >15, (ii) minimum depth ≥10 in blood and tumour, (iii) for a site to be scored as a loss of heterozygosity site, at least 20% of the reads that map to the site should contain the variant in the blood DNA; (iv) at least 10% of the reads should contain a variant in the tumour DNA for a site to be scored as a somatic variant site, (v) a variant site should have at least one read with the variant in each direction (to avoid strand bias), (vi) for every patient, clustered somatic mutations (two mutations in a 100-bp window) were removed, as these mutations were possibly generated as part of read misalignment error and (viii) somatic variants which are catalogued in the 1,000 Genomes, ESP genome database ( https://esp.gs.washington.edu/ ) with an allele frequency >0.01 were removed. If at a site both somatic and germline mutations were detected in our cohort, then the site was removed. Somatic mutations thus identified were annotated using the Annovar package and Oncotator module ( http://www.broadinstitute.org/ cancer/cga/oncotator) to infer the locations of the variants within the genes, effect of the mutation on the protein product and other features. All indels and recurrent substitutions were manually visualized and verified using IGV v2.1.25. Sequence data generated using GS-FLX Genome Sequencers, were converted to FASTQ format from SFF files by sffinfo (GS-FLX) and a Linux script developed by us. For data generated by Ion-torrent PGM, sequence reads were obtained in FASTQ format. The sequence data generated per run were evaluated by the same method described in the previous section. The GS-FLX derived FASTQ files were mapped to the human reference sequence hg19 (GRCh37) by SSAHA2 v2.5.5. PICARD v1.60 ( http://picard.sourceforge.net ) was used to remove PCR duplicates and combine SAM files from multiple runs. Pileup files were generated by SAMtools package. The pileup files of tumour and blood DNA from each patient were used to identify and verify putative variant sites using the base-by-base variant caller. For CNV, ASCAT 2.0 (alelle-specific copy number analysis of tumours) was used to identify regions of amplification and deletion using exported data from Illumina iScan Genome Studio software. Segments with mean LogR>0.15 were used to detect amplification segment and mean LogR<−0.2 were used to detect deletion. High-confidence CNV regions were annotated with NCBI refgene transcript database (hg19). Sequence BAM files for patients have been deposited in the European Genome-Phenome Archive under accession codes EGAS00001000249 and EGAS00001001028. Pathway analysis and other bioinformatics analyses PathScan module in GenomeMuSiC package [69] was used to identify somatic mutations enriched in annotated KEGG (Kyoto Encyclopedia of Genes and Genomes) AA metabolism pathway and other important mitogenic signalling pathways (PI3K, MAPK, JAK-STAT, WNT signalling). Only the loss-of-function mutations (non-synonymous, frame-shift and splice-site) were used in the PathScan analysis. Patients possessing a non-synonymous somatic mutation in a gene that overlapped with the Cancer Gene Census list (COSMIC Database) were identified. Similarly, the list of druggable genes [70] in mitogenic signalling pathways was searched for identifying the number of cancer genes mutated. Clinical and survival information for HNSCC and OSCC-GB patients included in the TCGA project were retrieved from the Synapse website https://www.synapse.org/#!Synapse:syn1446094 . Somatic mutation data of the corresponding patients for the AA metabolism pathway genes were downloaded from http://www.cbioportal.org/public-portal/ website. Analysis of TCGA-HNSCC functional proteomics data Custom search was done with 224 HNSCC patient IDs and AA metabolism pathway gene list on the cbioportal for cancer genomics ( http://www.cbioportal.org/public-portal/ ) for comparative analyses of mutation and reverse phase protein array data. Reverse phase protein array is a rapid high-throughput antibody-based technique to detect cellular protein levels; the procedure is very similar to western blotting. The custom analysis framework in cBioPortal produces a list of the significantly altered proteins based on their levels between patients with mutations in the list of mutated genes versus those with no mutations in genes on this list. A two-sided two sample Student’s t -test is used to detect significant protein alteration. Statistical tests Estimates of period of DFS for patients with mutAA genes versus patients with norAA genes were compared using the log-rank test. The survival probability distributions for both the groups were estimated using the Kaplan–Meier method. Two-sided statistical tests were used. Multivariate Cox proportional-hazards modelling was used to assess the possible prognostic significance of AAM pathway mutation on DFS. As all the patients were exposed to tobacco, tobacco use was not included as a covariate. In the Cox proportional-hazards analysis, age and number of somatic mutations were included as continuous variables, whereas all other factors were considered as categorical. P values for hazard ratios were calculated using the likelihood ratio test. P values <0.05 were considered to be significant. How to cite this article : Biswas, N. K. et al. Somatic mutations in arachidonic acid metabolism pathway genes enhance oral cancer post-treatment disease-free survival. Nat. Commun. 5:5835 doi: 10.1038/ncomms6835 (2014). Accession codes: Sequence BAM files for patients have been deposited in the European Genome-Phenome Archive under accession code EGAS00001001028.